Synthetic human cell fate regulation by protein-driven RNA switches Understanding how to control cell fate is crucial in biology, medical science and engineering. In this study, we introduce a method that uses an intracellular protein as a trigger for regulating human cell fate. The ON/OFF translational switches, composed of an intracellular protein L7Ae and its binding RNA motif, regulate the expression of a desired target protein and control two distinct apoptosis pathways in target human cells. Combined use of the switches demonstrates that a specific protein can simultaneously repress and activate the translation of two different mRNAs: one protein achieves both up- and downregulation of two different proteins/pathways. A genome-encoded protein fused to L7Ae controlled apoptosis in both directions (death or survival) depending on its cellular expression. The method has potential for curing cellular defects or improving the intracellular production of useful molecules by bypassing or rewiring intrinsic signal networks. In human cells, the specific regulation of target protein production at the post-transcriptional level has a significant role in determining cellular phenotypes, such as growth, proliferation, differentiation or programmed cell death (apoptosis) [1] , [2] , [3] . For instance, several studies comparing the amounts of expressed mRNAs and proteins in eukaryotic cells have demonstrated that expression of an mRNA only weakly correlates with that of the corresponding protein, indicating that protein expression is regulated not only at the transcriptional level but also at multiple post-transcriptional steps, including translational regulation and mRNA/protein degradation [1] , [4] , [5] , [6] . Although many synthetic methods have been reported for controlling transcription [7] , [8] , [9] , [10] , [11] , only a few methods for controlling translation have been reported so far [11] , [12] , [13] , [14] , [15] , [16] . A system that allows an endogenously expressed molecule such as a protein to control the expression level of a target gene would be especially advantageous. A method in which a specific protein produced in a cell can directly and quantitatively regulate the production of target protein(s) could be used to bypass or rewire intrinsic signalling networks and to construct novel cascades or feedback circuits for controlling cell functions ( Fig. 1a ) [17] , [18] . 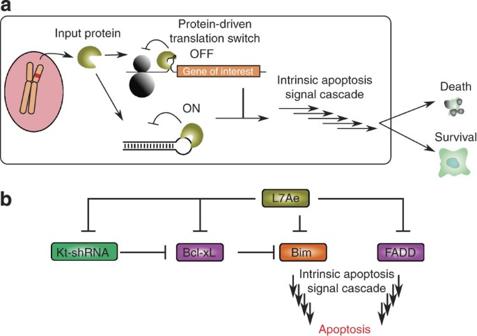Figure 1: Schematic diagram for regulation of cell death by protein-driven RNA ON/OFF switches. (a) Schematic representation of the outcome of this study. A protein encoded in genome drives translational switches and regulates intrinsic apoptosis signal cascade to control cell fate (death or survival). (b) Schematic diagram of the circuit connected to intrinsic apoptosis signal cascades regulated by the switches. Two distinct (mitochondria dependent and independent) apoptosis pathways controlled by L7Ae. L7Ae strictly regulates the production of apoptotic regulatory proteins (that is, Bcl-xL, Bim, FADD) involved in the complex intrinsic apoptosis signal cascades. Several steps of signal-transduction cascades and activation of a set of caspases are required to determine cell death. Figure 1: Schematic diagram for regulation of cell death by protein-driven RNA ON/OFF switches. ( a ) Schematic representation of the outcome of this study. A protein encoded in genome drives translational switches and regulates intrinsic apoptosis signal cascade to control cell fate (death or survival). ( b ) Schematic diagram of the circuit connected to intrinsic apoptosis signal cascades regulated by the switches. Two distinct (mitochondria dependent and independent) apoptosis pathways controlled by L7Ae. L7Ae strictly regulates the production of apoptotic regulatory proteins (that is, Bcl-xL, Bim, FADD) involved in the complex intrinsic apoptosis signal cascades. Several steps of signal-transduction cascades and activation of a set of caspases are required to determine cell death. Full size image Synthetic chimeric proteins have been used to rewire cell signalling pathways to control cell phenotype [19] , [20] , [21] . For example, signal transduction by the receptor tyrosine kinase ErbB2 was rewired by fusing SH2 or PTB domains of the adaptor proteins Grb2 and ShcA to the death effector domain of FADD (Fas-Associated protein with Death Domain) [22] . In this system, the chimeric adaptors relayed the signal from epidermal growth factor (EGF) to the caspase 8-dependent apoptotic pathway to induce cell death. However, the controllable signalling pathways are limited to those using the available adaptor proteins. It also remains unknown whether a protein expressed in cells can be used as a triggering signal for regulating the expression of a desired protein in these systems. In this study, we report advanced protein-driven translational regulatory ON/OFF systems for controlling the fate of human cells ( Fig. 1a,b ). The design of the OFF system was based on our previously reported translational repression system [15] consisting of an archaeal ribosomal protein, L7Ae, and its binding RNA motif, box C/D kink-turn (Kt) [23] . In the OFF system, L7Ae expressed in human cells directly and quantitatively inhibits the translation of a target gene. A new translational activation (ON) system triggered by L7Ae has also been developed for regulating the processing of short hairpin RNAs (shRNAs). We were able to efficiently control apoptosis in human cells with each system individually and in combination. In conclusion, we have shown here a new approach for determining human cell fate by using a specific genome-encoded protein that serves as an index of the cellular environment ( Fig. 1a ). Quantitative translational repression in living cells We first investigated whether we could observe quantitative translational control by L7Ae in individual living cells. Two plasmids were constructed: pKt- GFP -I- CFP , in which the mRNA contains the box C/D Kt motif incorporated upstream of the AUG codon of the EGFP coding sequence, and pdKt- GFP -I- CFP , which contains a defective Kt motif. For pKt- GFP -I- CFP , EGFP production is under the control of the expression of L7Ae because of the interaction between L7Ae and the Kt motif. As ECFP production from IRES is independent of L7Ae, the ratio of the EGFP and ECFP signals indicates the level of translational repression ( Supplementary Fig. S1a ). The red fluorescent protein (AsRed2) was fused with L7Ae (AsRed2-L7Ae) to quantify the expression level of L7Ae for normalization of the data. Overall translational repression efficiencies across the entire population of cells confirmed that the OFF system is highly efficient and selective ( Supplementary Fig. S1b ). We next analysed the efficiency in individual cells. The results indicate that EGFP production from the Kt -GFP -I- CFP mRNA was repressed quantitatively and selectively in individual cells depending on the expression level of L7Ae ( Supplementary Fig. S1c ). Thus, we conclude that the efficiency of translational regulation corresponds to the expression level of the input L7Ae protein. Reprogramming cell death pathways with the OFF system The OFF system was applied for controlling human cell fate by modulating the translation of apoptosis regulatory proteins ( Fig. 1b ). The mitochondrial-dependent apoptosis pathways were used to control intrinsic apoptosis pathways ( Fig. 1b , Bcl-xL/Bim-dependent pathways) because the balance between proapoptotic (that is, Bim) and antiapoptotic (that is, Bcl-xL) Bcl-2 family proteins determines cell fate [24] . Namely, the control of apoptosis pathways by gene regulation requires strict expression balance between pro- and antiapoptotic proteins [25] . For instance, the leaky expression of a proapoptotic gene makes it difficult to suppress apoptosis, as it amplifies apoptosis signals by positive feedback mechanism [26] , [27] . To control apoptosis by L7Ae, we constructed the following three plasmids: pKt- Bcl-xL -I- GFP (an antiapoptotic agent), pdKt- Bcl-xL -I- GFP (a negative control plasmid containing a defective Kt) and a plasmid encoding Bim (p Bim , a proapoptotic agent) ( Fig. 2a , Supplementary Fig. S2 ). Western blot analysis showed that L7Ae expressed in HeLa cells efficiently represses the expression of Bcl-xL from pKt- Bcl-xL -I- GFP ( Fig. 2b , lane 5), but has no effect on the defective Kt mutant, pdKt- Bcl-xL -I- GFP ( Fig. 2b , lane 7). Flow cytometric analysis confirmed that expression of Bcl-xL from pKt- or pdKt- Bcl-xL -I- GFP efficiently repressed Bim-induced apoptosis in cells ( Fig. 2c , lane 2 versus lane 3 or 5). In addition, L7Ae triggered an apoptosis-inducing signal in the corresponding cells by promoting the translational regulation of Bcl-xL. Expression of L7Ae induced apoptosis specifically in cells containing both p Bim and pKt- Bcl-xL -I- GFP ( Fig. 2c , lane 4; Supplementary Fig. S3 ). An analysis of cell morphology confirmed that L7Ae induced apoptosis by repressing Bcl-xL expression in target cells ( Fig. 2d , left, middle picture), whereas the normal phenotype was observed for cells containing the control plasmid ( Fig. 2d , right, middle picture). Thus, L7Ae expressed in cells containing Kt- Bcl-xL mRNA induces apoptosis by repressing the expression of Bcl-xL. 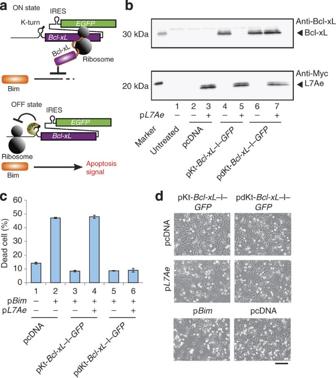Figure 2: Regulation of the apoptosis pathway using the OFF system. (a) Schematic illustration of the ON/OFF states of the switch. In cells that do not express L7Ae, translated Bcl-xL protein binds to Bim to prevent apoptosis (ON state). L7Ae represses translation of Bcl-xL, and the apoptosis signal from Bim can proceed (OFF state). (b) Western blotting analysis of Bcl-xL expression in HeLa cells co-transfected withpL7Aeand p(d)Kt-Bcl-xL-I-GFP. Bcl-xL and L7Ae were detected using anti-Bcl-xL and anti-myc antibodies, respectively. (c) Flow cytometric analysis performed 24 h after co-transfection with pBimand the plasmids described inb. The data are presented as the mean±s.d. of triplicate experiments. (d) Phase microscopic images of the cells analysed inc. A scale bar represents 200 μm. Figure 2: Regulation of the apoptosis pathway using the OFF system. ( a ) Schematic illustration of the ON/OFF states of the switch. In cells that do not express L7Ae, translated Bcl-xL protein binds to Bim to prevent apoptosis (ON state). L7Ae represses translation of Bcl-xL, and the apoptosis signal from Bim can proceed (OFF state). ( b ) Western blotting analysis of Bcl-xL expression in HeLa cells co-transfected with pL7Ae and p(d)Kt- Bcl-xL -I- GFP . Bcl-xL and L7Ae were detected using anti-Bcl-xL and anti-myc antibodies, respectively. ( c ) Flow cytometric analysis performed 24 h after co-transfection with p Bim and the plasmids described in b . The data are presented as the mean±s.d. of triplicate experiments. ( d ) Phase microscopic images of the cells analysed in c . A scale bar represents 200 μm. Full size image To demonstrate the modularity of the OFF switch, we constructed an alternative system to direct cell fate towards survival by regulating a mitochondria-independent apoptotic pathway ( Fig. 1b , FADD-dependent pathway). The expression of FADD has a critical role in inducing apoptosis in this pathway ( Fig. 1b , right; Supplementary Fig. S4 ) [28] . We attempted to downregulate apoptosis by repressing the production of FADD with the L7Ae system ( Supplementary Fig. S5a ). L7Ae downregulated apoptosis effectively and specifically by repressing translation of FADD derived from pKt- FADD plasmid ( Supplementary Fig. S5b–f ). These results indicate that by repressing the expression of either anti- or proapoptotic proteins, the OFF system can steer the apoptosis pathway towards death or survival, respectively. Synthetic translational activation of a target mRNA Like the OFF system, the protein-triggered translational activation system (ON system) should work as a 'protein–protein information converter' that transmits information carried by an input protein (for example, L7Ae) to the desired output protein (for example, Bcl-xL). Such converters are useful for bypassing intrinsic cell signalling pathways or constructing synthetic signalling pathways ( Fig. 1 ) [19] , [20] . To construct the ON system in human cells, we designed and constructed a synthetic shRNA [29] , [30] , [31] containing an siRNA and the Kt motif in its stem and loop regions, respectively ( Figs 1 and 3a; Supplementary Fig. S6 ). We will refer to this construct as Kt-shRNA. In this system, the Kt-shRNA is designed to result in specific degradation of a target mRNA by RNA interference (RNAi). Conversely, cellularly expressed L7Ae binding to Kt-shRNA is expected to interfere with Dicer-dependent cleavage of the shRNA, resulting in L7Ae-controlled protection of the target mRNA ( Fig. 3a ). 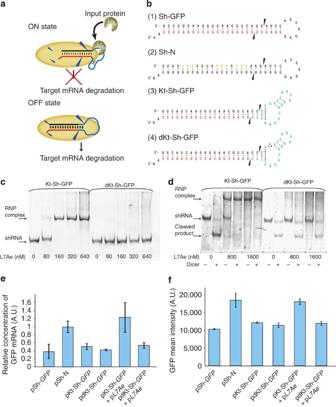Figure 3: Protein-driven ON system. (a) Schematic illustration of the ON/OFF states. (b) Sh-GFPtargeting theEGFPgene. The sequence in red is complementary toEGFPmRNA (1). Sh-N was designed not to knockdown any gene and encodes a stop codon (in yellow) in every frame (2). We designed Kt-Sh-GFPby incorporating the Kt motif into the loop region of the Sh-GFP(3). dKt-Sh-GFPis defective for the Kt motif in the loop region (4). (c) Determination of the binding affinity of Kt-Sh-GFP(40 nM) and L7Ae (0–640 nM) using the gel shift assay. Kt-Sh-GFPand L7Ae were mixed in transfection buffer, Opti-MEMI (Invitrogen), and separated in the gel shift assay. (d) The specific binding of Kt and L7Ae repressed Dicer cleavage activity for Kt-Sh-GFP. In the presence of L7Ae, Kt-Sh-GFPand L7Ae formed an RNP complex and prevented Dicer cleavage, yet the mutant dKt-Sh-GFPwas still cleaved. (e) The relative concentration ofEGFPmRNA. (f) The intensity of EGFP fluorescence in HeLa cells stably expressing EGFP (HeLa-GFP). These indicated that L7Ae-specific binding to Kt-Sh-GFP repressed the knock down function of Kt-Sh-GFPand, as a result, inhibitedEGFPmRNA degradation and reactivated EGFP expression in HeLa-GFP cells. Foreandf, the error bar indicates the standard deviation of three independent samples. Sh-GFPand Sh-N were used for positive and negative controls of EGFP knockdown, respectively. Figure 3: Protein-driven ON system. ( a ) Schematic illustration of the ON/OFF states. ( b ) Sh- GFP targeting the EGFP gene. The sequence in red is complementary to EGFP mRNA (1). Sh-N was designed not to knockdown any gene and encodes a stop codon (in yellow) in every frame (2). We designed Kt-Sh- GFP by incorporating the Kt motif into the loop region of the Sh- GFP (3). dKt-Sh- GFP is defective for the Kt motif in the loop region (4). ( c ) Determination of the binding affinity of Kt-Sh- GFP (40 nM) and L7Ae (0–640 nM) using the gel shift assay. Kt-Sh- GFP and L7Ae were mixed in transfection buffer, Opti-MEMI (Invitrogen), and separated in the gel shift assay. ( d ) The specific binding of Kt and L7Ae repressed Dicer cleavage activity for Kt-Sh- GFP . In the presence of L7Ae, Kt-Sh- GFP and L7Ae formed an RNP complex and prevented Dicer cleavage, yet the mutant dKt-Sh- GFP was still cleaved. ( e ) The relative concentration of EGFP mRNA. ( f ) The intensity of EGFP fluorescence in HeLa cells stably expressing EGFP (HeLa-GFP). These indicated that L7Ae-specific binding to Kt-Sh-GFP repressed the knock down function of Kt-Sh- GFP and, as a result, inhibited EGFP mRNA degradation and reactivated EGFP expression in HeLa-GFP cells. For e and f , the error bar indicates the standard deviation of three independent samples. Sh- GFP and Sh-N were used for positive and negative controls of EGFP knockdown, respectively. Full size image Before performing cell fate control experiments, we confirmed that the Kt-shRNA, which targeted the EGFP gene for RNAi (Kt-Sh- GFP ; Fig. 3b ), interacted specifically with recombinant L7Ae in vitro ( Fig. 3c ). We observed that the catalytic activity of Dicer was efficiently blocked by the RNA–protein (RNP) interaction ( Fig. 3d ). Two shRNA-coding plasmids, pKt-Sh- GFP and the corresponding negative control plasmid, pdKt-Sh- GFP , containing a defective Kt, were tested to show that they effectively downregulated the expression of EGFP at both the protein and the mRNA levels ( Figs 3e,f ). As expected, L7Ae expressed in HeLa cells could upregulate EGFP expression by binding to pKt-Sh- GFP , but it did not affect the downregulation of EGFP expression by pdKt-Sh- GFP ( Fig. 3f ). To regulate cell fate, we prepared three shRNA-coding plasmids that targeted the Bcl-xL gene: pSh- Bcl-xL (positive control), pKt-Sh- Bcl-xL and pdKt-Sh- Bcl-xL ( Fig. 4a ). L7Ae selectively inhibited the activity of Dicer on Kt-Sh- Bcl-xL RNA in vitro , but not on dKt-Sh- Bcl-xL RNA ( Fig. 4b ). Western blotting showed that transfection of pKt-Sh- Bcl-xL or pdKt-Sh- Bcl-xL repressed expression of Bcl-xL in cells after 24 h as effectively as the positive control, pSh- Bcl-xL ( Fig. 4c , lanes 7 and 8). Conversely, L7Ae protected the expression of Bcl-xL from repression by pKt-Sh- Bcl-xL selectively and effectively ( Fig. 4c , lane 5). The results indicate that the interaction between L7Ae and Kt-shRNA inhibits RNAi activity, which results in translation of the protected target mRNA. 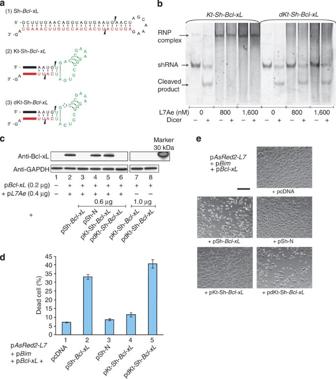Figure 4: Using the ON system to control cell fate. (a) Targeting theBcl-xLgene with shRNAs containing a loop (1), Kt (2, green) and dKt (3, green). The sequence in red is the complementary strand of a region ofBcl-xLmRNA. The cleavage sites of the Dicer enzyme are indicated by arrowheads. (b) The Dicer cleavage assayin vitro. (c) Western blotting analysis of Bcl-xL using the L7Ae-K-turn ON switch in cells. (d) Flow cytometric analysis of cell death performed 24 h after co-transfection with pAsRed2-L7Ae, pBcl-xL, pBimand the corresponding pshRNA. The data are presented as the mean±s.d. of triplicate experiments. (e) Analysis of the morphology of the cells indby phase microscopy. A scale bar represents 200 μm. Figure 4: Using the ON system to control cell fate. ( a ) Targeting the Bcl-xL gene with shRNAs containing a loop (1), Kt (2, green) and dKt (3, green). The sequence in red is the complementary strand of a region of Bcl-xL mRNA. The cleavage sites of the Dicer enzyme are indicated by arrowheads. ( b ) The Dicer cleavage assay in vitro . ( c ) Western blotting analysis of Bcl-xL using the L7Ae-K-turn ON switch in cells. ( d ) Flow cytometric analysis of cell death performed 24 h after co-transfection with p AsRed2-L7Ae , p Bcl-xL , p Bim and the corresponding pshRNA. The data are presented as the mean±s.d. of triplicate experiments. ( e ) Analysis of the morphology of the cells in d by phase microscopy. A scale bar represents 200 μm. Full size image The ON system was used to control cell fate by activating Bcl-xL translation in the presence of L7Ae. Flow cytometric ( Fig. 4d , lane 4) and cell morphology ( Fig. 4e , left, bottom picture) analyses showed that the system repressed Bim-induced apoptosis by activating Bcl-xL expression ( Fig. 1b ). Taken together, the data indicate that the synthetic translational ON and OFF systems can each control cell fate in the desired direction (death or survival) by modulating translation of the target mRNAs. Simultaneous control of cell fate by both ON and OFF systems We next attempted to simultaneously repress the translation of one mRNA and activate expression of a second mRNA in human cells by using L7Ae. Plasmids encoding AsRed2, designed to serve as a repressible gene (AsRed2-OFF), and EGFP, designed to serve as an activating gene (EGFP-ON), were constructed. L7Ae expression simultaneously and selectively repressed the translation of AsRed2 and activated EGFP, which we confirmed by flow cytometry ( Figs 5a,b ) and fluorescence microscopy ( Fig. 5c ). The results indicate that a single protein simultaneously represses and activates translation of two different mRNAs in human cell. 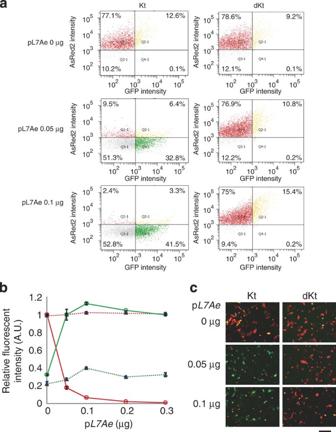Figure 5: Simultaneous translational repression and activation of two fluorescent proteins by synchronized ON/OFF switches. (a) Simultaneous translational activation and repression of EGFP and AsRed2 by synchronized ON/OFF switches. The fluorescence intensity of the transfected cells was analysed by flow cytometry. These dot plot data correspond to the fluorescent microscopic images inFigure 5c. (b) Flow cytometric analysis of the simultaneous regulation of EGFP-ON and AsRed2-OFF switches by L7Ae. The efficiencies of translation were normalized to control translational rates in the absence of pL7Ae(AsRed2-OFF) or in the presence of 0.3 μg of pL7Ae(EGFP-ON). The results are presented as the mean±s.d. of triplicate experiments. Green solid line with circles; EGFP relative intensity (Kt), green dashed line with triangles; EGFP relative intensity (dKt), red solid line with circles; AsRed2 relative intensity (Kt), red dashed line with triangles; AsRed2 relative intensity (dKt). (c) Merged fluorescent microscopic images of cells that contained EGFP-ON and AsRed2-OFF switches. A scale bar represents 200 μm. Figure 5: Simultaneous translational repression and activation of two fluorescent proteins by synchronized ON/OFF switches. ( a ) Simultaneous translational activation and repression of EGFP and AsRed2 by synchronized ON/OFF switches. The fluorescence intensity of the transfected cells was analysed by flow cytometry. These dot plot data correspond to the fluorescent microscopic images in Figure 5c . ( b ) Flow cytometric analysis of the simultaneous regulation of EGFP-ON and AsRed2-OFF switches by L7Ae. The efficiencies of translation were normalized to control translational rates in the absence of p L7Ae (AsRed2-OFF) or in the presence of 0.3 μg of p L7Ae (EGFP-ON). The results are presented as the mean±s.d. of triplicate experiments. Green solid line with circles; EGFP relative intensity (Kt), green dashed line with triangles; EGFP relative intensity (dKt), red solid line with circles; AsRed2 relative intensity (Kt), red dashed line with triangles; AsRed2 relative intensity (dKt). ( c ) Merged fluorescent microscopic images of cells that contained EGFP-ON and AsRed2-OFF switches. A scale bar represents 200 μm. Full size image The combined use of the ON/OFF systems was tested for controlling apoptotic pathways in human cells. The OFF and ON switches were designed to repress proapoptotic Bim (Bim-OFF) and to activate antiapoptotic Bcl-xL (Bcl-xL-ON), respectively ( Fig. 1b ). As expected, L7Ae simultaneously repressed Bim expression and activated Bcl-xL expression to successfully modulate apoptosis ( Fig. 6a , lane 3; Fig. 6b , top left). We were able to unidirectionally control human cell fate by appropriately connecting the two systems to the existing signalling networks. 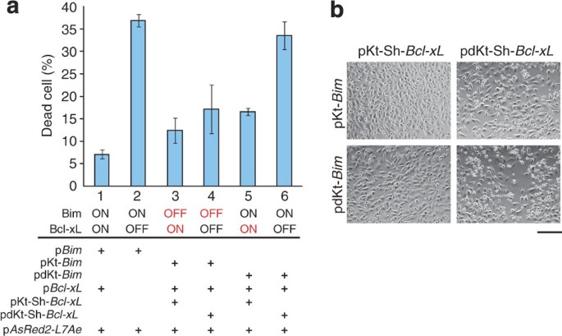Figure 6: Simultaneous translational repression and activation of apoptotic proteins by synchronized ON/OFF switches. (a) Regulation of apoptosis by the synchronized Bcl-xL-ON and Bim-OFF switches. Cells that contain Kt-Bimand Kt-Sh-Bcl-xLwere protected from Bim-induced apoptosis by expressing L7Ae (lane 3), whereas cells that contain dKt-Bimand dKt-Sh-Bcl-xLinduced apoptosis (lane 6). The cells were analysed by using flow cytometry. Kt-ON/OFF switches are shown in red. The results are presented as the mean±s.d. of triplicate experiments. (b) Cell morphology analysis ofFigure 6aby phase microscopy. Scale bars represent 200 μm. Figure 6: Simultaneous translational repression and activation of apoptotic proteins by synchronized ON/OFF switches. ( a ) Regulation of apoptosis by the synchronized Bcl-xL-ON and Bim-OFF switches. Cells that contain Kt- Bim and Kt-Sh- Bcl-xL were protected from Bim-induced apoptosis by expressing L7Ae (lane 3), whereas cells that contain dKt- Bim and dKt-Sh- Bcl-xL induced apoptosis (lane 6). The cells were analysed by using flow cytometry. Kt-ON/OFF switches are shown in red. The results are presented as the mean±s.d. of triplicate experiments. ( b ) Cell morphology analysis of Figure 6a by phase microscopy. Scale bars represent 200 μm. Full size image Control of apoptosis by a protein encoded in genome Finally, we investigated to see whether a protein of interest encoded in the genome quantitatively controls apoptosis pathways as a function of the protein expression. The insertion of L7Ae into the genome allows us to use L7Ae as a molecular tag for a protein of interest. As a pilot system, we attempted to quantitatively regulate apoptosis by controlling the expression level of an input protein (L7Ae-tagged red fluorescent protein: DsRed-L7Ae) encoded in the genome. A stable cell line (T-REx HeLa) was used for the conditional expression of DsRed-L7Ae in the presence of tetracycline. Western blotting analysis confirmed that the repression of Bcl-xL production depends quantitatively on the expression of DsRed-L7Ae ( Fig. 7a ). Moreover, apoptosis of the target cells was induced by the expression of DsRed-L7Ae in a dose-dependent manner ( Fig. 7b ). We were also able to repress apoptosis by controlling FADD expression by using DsRed-L7Ae expressed from the genome ( Supplementary Fig. S7 ). Thus, it seems certain that a specific protein encoded in the genome can drive the translational regulatory systems to control cell fate. 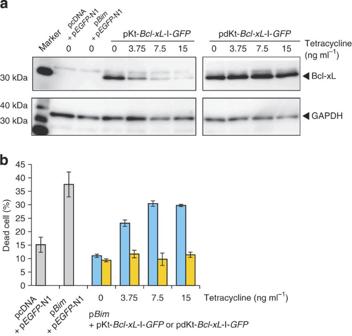Figure 7: Quantitative regulation of apoptosis by L7Ae-DsRedMprotein derived from DNA integrated into genome. (a) Western blotting analysis of cell lysates 24 h after transfection with pKt-Bcl-xL-I-GFP(or pdKt-Bcl-xL-I-GFP) and pBimin the absence or presence of tetracycline (0–15 ng ml−1) using anti-Bcl-xLantibody. (b) Flow cytometric analysis of the same cells. Cells positive for EGFP and Pacific Blue were considered dead. Blue column, Kt; yellow column, dKt. The results are presented as the mean±s.d. of triplicate experiments. Figure 7: Quantitative regulation of apoptosis by L7Ae-DsRed M protein derived from DNA integrated into genome. ( a ) Western blotting analysis of cell lysates 24 h after transfection with pKt- Bcl-xL -I- GFP (or pdKt- Bcl-xL -I- GFP ) and p Bim in the absence or presence of tetracycline (0–15 ng ml −1 ) using anti- Bcl-xL antibody. ( b ) Flow cytometric analysis of the same cells. Cells positive for EGFP and Pacific Blue were considered dead. Blue column, Kt; yellow column, dKt. The results are presented as the mean±s.d. of triplicate experiments. Full size image In this study, we have shown that the RNP switch containing the L7Ae–Kt RNP interaction motif enables the control of human cell phenotype. A specific protein (L7Ae or L7Ae-tagged protein of interest) expressed in cells repressed and activated translation of specific mRNAs coding the proteins (that is, Bcl-xL, Bim, FADD) involved in the signal-transduction cascades. Moreover, the protein-driven ON/OFF systems can control the intrinsic apoptosis signalling circuits (that is, mitochondria-dependent and -independent apoptosis pathways) to determine cell phenotype (cell death) ( Figs 1a,b ). The strict apoptotic control in this study is attributed to the efficient gene regulation by the RNP switches ( Figs 2 , 4 and 5; Supplementary Fig. S1 ), indicating that it serves as a versatile switch in other applications. As a pilot system, a protein of interest fused to L7Ae that is integrated in the genome quantitatively controlled apoptosis pathways ( Fig. 7 , Supplementary Fig. S7 ), indicating that it is feasible to construct a system for controlling phenotype of cell as a function of changes in the cellular environment (that is, expression of a specific protein) in general ( Fig. 1a ). Small molecules, such as tetracycline or theophylline, have been used as triggers for synthetic translational regulation. The most popular system using RNA aptamers for theophylline has been used to determine the activation (ON) or repression (OFF) of gene expression in bacteria and yeast cells [12] , [32] , [33] . Efficient synthetic genetic switches triggered by the small molecule have also been constructed by combining RNAi regulatory systems with repressor proteins in mammalian cells [34] . These methods are versatile and universally applicable. However, the control of cell function depending on the expression level of a particular gene of interest is extremely difficult by using a small molecule as an input signal. Our protein-driven RNP switches are advantageous for the use in the signal-transduction cascades because protein molecules can be used as both input and output signals that is impossible for small molecule-based systems. For instance, an L7Ae–Kt interaction-based translational auto-feedback system could allow the sophisticated control of protein production depending on the cellular environment in a manner similar to naturally occurring translational feedback systems [35] . In our preliminary experiments, cellularly expressed L7Ae modulated its own translation level by binding to the Kt motif of the mRNA (Stapleton, J.A. et al ., unpublished data). Thus, the ON/OFF switch could serve as a unique tool for accurately controlling cell fate because expression levels from particular mRNAs can vary in a spatiotemporal manner [36] to induce a variety of cell phenotypes [37] . Proteins other than L7Ae are potentially usable as new regulators for the system as follows: (1) The L7Ae protein could be used to tag other proteins of interest, and (2) a variety of RNA–protein binding motifs, including naturally occurring and in vitro -selected RNA aptamers, could be used for constructing new translational switches [38] . RNP interaction motifs can be seen as a new molecular resource for constructing libraries of interoperable components and modules [39] . Accordingly, development of a set of new RNP interaction motifs could be useful for next-generation and real-world application of synthetic gene networks [9] , [15] , [39] , [40] . For instance, in vitro -selected aptamers could directly sense the expression of target marker proteins (for example, Bcl-xL, the expression level of which is known to be upregulated in certain cancer cells), and control the expression of the desired output proteins (for example, activation of a cell killer gene; Supplementary Fig. S8 ). Thereby, the switch could induce apoptosis in the target cancer cells. As another example, our RNP switches could be used for controlling the expression of multiple genes to produce useful molecules [40] , [41] , because the switches simultaneously repress and activate translation of different mRNAs as a function of the expression of specific proteins in living cells. The combined use of our RNP switch and other established regulatory systems based on transcriptional control [42] , modular engineering of chimeric proteins [19] , [43] or small molecule-based riboswitches [12] , [32] , [33] , [44] , [45] , [46] could further enhance the efficacy of the system when multiple actions are required to assure the outcome. Cell culture and treatments HeLa cells and HeLa-GFP cells were cultured at 37 °C in 5% CO 2 in DMEM/F-12 (Dulbecco's modified Eagle's medium: Nutrient Mixture F-12) 1:1 mixture (Invitrogen), supplemented with an antibiotic solution (A5955, Sigma) and 10% calf bovine serum (CBS, MP Bioscience) or fetal bovine serum (CCB). HeLa-GFP cells were additionally supplemented with 50 μg ml −1 of Hygromycin B (Invitrogen). The DsRed-L7Ae-inducible cell line (T-REx HeLa-DsRed-L7Ae) was established previously [15] as follows. T-REx HeLa cells (Invitrogen), cultured in fresh medium supplemented with 10% CBS (#2001H, MP Biomedicals), were transfected with pcDNA4/TO/DsRed-L7 containing the tetracycline-regulatable promoter and the DsRed M -L7Ae gene. After 24 h, the medium was replaced with fresh medium supplemented with 10% CBS, 5 μg ml −1 blasticidin (Invivogen) and 100–200 μg ml −1 zeocin (Invitrogen) for selection. The cells were cultured in selective medium every 3–4 days until foci could be identified. The selected cells were cloned using a cell sorter (FACS Aria, BD Biosciences). The clone exhibiting the highest expression level of DsRed M -L7Ae in the presence of Tet was confirmed by western blotting and named H5. The H5 cells were cultured in DMEM/F-12 supplemented with 10% CBS, 5 μg ml −1 blasticidin and 150 μg ml −1 zeocin. Transfection Cells were plated into appropriate multi-well plates. After 1 day, the 70–90% confluent cells were transfected with plasmids using Lipofectamine 2000 according to the standard protocols included in the Lipofectamine 2000 kit (Invitrogen). After 4 h of transfection, the medium was replaced with fresh medium if needed. DNA preparation All DNA templates and primers were purchased from Hokkaido System Science or Gene Design. PCR amplifications were carried out using Ex Taq DNA polymerase (TAKARA BIO) or KOD-PLUS-DNA polymerase (TOYOBO). Apoptosis assay Apoptotic and dead cells were stained with Pacific Blue-labelled annexin V according to the standard protocols of the Vybrant Apoptosis Assay Kit #14 (Invitrogen). Dead cells were additionally stained by 7-AAD (Invitrogen) if needed. The stained cells were analysed on a FACS Aria. A 405 nm semiconductor laser was used for excitation of the Pacific Blue, and a 488 nm laser was used for EGFP, DsRed M , AsRed2 and 7-AAD. The 450/40 nm, 530/30 nm and 695/40 nm bandpass filters were used for collection of the fluorescent signals from Pacific Blue, EGFP and 7-AAD, respectively. When EGFP and DsRed M (or AsRed2) were expressed simultaneously, a 695/40 nm bandpass filter was used for the signals from DsRed M (or AsRed2); otherwise, a 616/23 nm bandpass filter was used. The remaining cells were collected and stored at −20 °C for analysis by western blotting, if needed. Translational repression assay of apoptosis regulatory proteins For western blotting analysis of repression of Bcl-xL in cells, HeLa cells (1×10 5 per well) were seeded onto 12-well plates. p L7Ae (0.4 μg) and pKt- Bcl-xL -I- GFP (or dKt- Bcl-xL -I- GFP , 0.2 μg) were co-transfected into HeLa cells. A blank plasmid, pcDNA that stands for pcDNA3.1-MycHisA (Invitrogen), was used as a control. Twenty-four hours after transfection, the cells were collected by trypsinization and Bcl-xL was detected using an anti-Bcl-xL antibody. For analysis of apoptosis regulated by Bcl-xL and Bim, HeLa cells were co-transfected as described above, except that the cells were additionally co-transfected with 0.2 μg of p Bim . After 24 h, collected cells were stained by Pacific Blue-labelled annexin V and 7-AAD and analysed on a FACS Aria. Only EGFP-positive cells were analysed to eliminate debris, dust or untransfected cells. Pacific Blue-positive cells were considered dead. For quantitative regulation of apoptosis, the DsRed-L7Ae-inducible cell line (3×10 5 per well) was used instead of HeLa cells. Cells were co-transfected with 0.4 μg of pKt- Bcl-xL -I- GFP (or dKt- Bcl-xL -I- GFP ) and 0.4 μg of p Bim using 2 μl Lipofectamine 2000. After 4 h, expression of DsRed-L7Ae was induced by tetracycline (Invitrogen) at 0–15 ng ml −1 . After 24 h, the cells were stained by Pacific Blue-labelled annexin V and analysed on the FACS Aria. To confirm proapoptotic activities of FADD and its pathway, DsRed-L7Ae-inducible cell lines (3×10 5 per well) were seeded onto 12-well plates. The cells were co-transfected with 0.9 μg of pKt- FADD and 0.4 μg of p EGFP -N1 in the presence or absence of 20 μM of Z-V-FMK (Sigma). For analysis of apoptosis regulated by FADD, HeLa cells (5×10 5 per well) were seeded onto six-well plates. The cells were co-transfected with 0.5 μg of pKt- FADD (or pdKt- FADD ) and 1 μg of p L7Ae and collected after 24 h. Expression of FADD in the cells was detected by western blotting using an anti-c-Myc antibody. To eliminate untransfected cells, cells were additionally co-transfected with 0.2 μg of p EGFP -N1 for flow cytometric analysis. The collected cells were stained by Pacific Blue-labelled annexin V and 7-AAD and subjected to flow cytometric analysis. Pacific Blue-positive cells were considered dead. Dicer-dependent shRNA in vitro cleavage assay Kt-Sh- Bcl-xL or dKt-Sh- Bcl-xL (40 nM) and the purified L7Ae protein (0, 800 or 1,600 nM) were mixed with 1 μl of 10 mM ATP, 0.5 μl of 50 mM MgCl 2 , 4 μl of Dicer Reaction Buffer (Genlantis), 2 μl of 0.5 U μl −1 Recombinant Human Dicer Enzyme (Genlantis), and water (up to 10 μl). The mixtures were incubated at 37 °C for 14 h and incubation was stopped with 2 μl of Dicer Stop Solution. The mixtures were separated by 15% native PAGE at 4 °C for 50 min and the gel was stained with SYBER-Green (TAKARA BIO). The fluorescence of the stained RNA was detected by FLA-7000 (Fujifilm) ( Fig. 4b ). Kt-Sh- GFP and dKt-Sh- GFP were also analysed using the above procedure ( Fig. 3d ). Translational activation assay of Bcl-xL To examine the re-activation efficiency of Bcl-xL translation triggered by Kt-L7Ae binding, we co-transfected HeLa cells (3×10 5 per well) grown for 1 day in 12-well plates with p Bcl-xL , p(d)Kt-Sh- Bcl-xL and p L7Ae using 2.5 μl of Lipofectamine 2000. Twenty-four hours after transfection, Bcl-xL was quantified by western blotting analysis. To examine the efficiency of cell fate determination through the control of Bcl-xL translation triggered by Kt-L7Ae binding, we co-transfected HeLa cells (0.5×10 5 per well) grown for 1 day in 24-well plates with 0.2 μg of p Bim , 0.2 μg of p Bcl-xL , 0.3 μg of p(d)Kt-Sh- Bcl-xL and 0.2 μg of p AsRed2-L7Ae using 1.25 μl of Lipofectamine 2000. Twenty-four hours after transfection, following a cell morphology analysis, the cells and medium were collected and stained with Pacific Blue-labelled annexin V as described in the apoptosis assay. The populations of apoptotic and dead cells, which exhibited high fluorescence intensity of Pacific Blue, were analysed using a flow cytometer. To eliminate abnormal cells, those cells whose fetal calf serum and Superconducting Super Collider signal scopes were identical to those of untreated HeLa cells were selected for the calculation of mean intensities. The red fluorescence of AsRed2-L7 was used as a marker for co-transfected cells. pSh- Bcl-xL and pSh-N were used for positive and negative controls of Bcl-xL knockdown, respectively. Synchronized control of ON/OFF translational switches For the synchronized control of AsRed2-OFF and EGFP-ON switches triggered by Kt-L7Ae binding in the same cells, we co-transfected HeLa cells (0.8×10 5 per well) grown for 1 day in 24-well plates with 0, 0.05, 0.1, 0.2, 0.3 μg of pL7Ae and pcDNA (total amount 0.3 μg), 0.1 μg of pEGFP, 0.3 μg of p(d)Kt-Sh-GFP and 0.1 μg of p(d)Kt-AsRed2-I-CFP with 1.5 μl of Lipofectamine 2000. Transfection for fluorescent microscopic analysis was performed similarly, but with the replacement of p(d)Kt-AsRed2-I-CFP with p(d)Kt-AsRed2. Twenty-four hours after transfection, cells and medium were collected and re-suspended in medium. To measure the EGFP and AsRed2 fluorescence intensities, the CFP-expressing cells (as a positive control for the transfected cells) were analysed by a flow cytometer. The abnormal cells were eliminated as described in the translational activation assay. For the simultaneous control of Bim repression and Bcl-xL activation by mixing the Kt-L7Ae OFF and ON switches, we co-transfected HeLa cells (1.0×10 5 per well) grown for 1 day in 24-well plates with 0.2 μg of pBcl-xL, 0.2 μg of pAsRed2-L7Ae, 0.2 μg of p(d)Kt-Bim and 0.3 μg of p(d)Kt-Sh-Bcl-xL (the total amount of transfected plasmids was compensated with pcDNA up to 0.9 μg) with 1.25 μl of Lipofectamine 2000. Twenty-four hours after transfection, following cell morphology analysis, the cells and medium were collected and stained with Pacific Blue-labelled annexin V as described in the apoptosis assay. The populations of apoptotic and dead cells, which exhibited high fluorescence intensity of Pacific Blue, were analysed using a flow cytometer. The red fluorescence of AsRed2-L7 was used as a marker for co-transfected cells. How to cite this article: Saito, H. et al . Synthetic human cell fate regulation by protein-driven RNA switches. Nat. Commun. 2:160 doi: 10.1038/ncomms1157 (2011).